Polycomb dysregulation in gliomagenesis targets aZfp423-dependent differentiation network Malignant gliomas constitute one of the most significant areas of unmet medical need, owing to the invariable failure of surgical eradication and their marked molecular heterogeneity. Accumulating evidence has revealed a critical contribution by the Polycomb axis of epigenetic repression. However, a coherent understanding of the regulatory networks affected by Polycomb during gliomagenesis is still lacking. Here we integrate transcriptomic and epigenomic analyses to define Polycomb-dependent networks that promote gliomagenesis, validating them both in two independent mouse models and in a large cohort of human samples. We find that Polycomb dysregulation in gliomagenesis affects transcriptional networks associated with invasiveness and de-differentiation. The dissection of these networks uncovers Zfp423 as a critical Polycomb-dependent transcription factor whose silencing negatively impacts survival. The anti-gliomagenic activity of Zfp423 requires interaction with the SMAD proteins within the BMP signalling pathway, pointing to a novel synergic circuit through which Polycomb inhibits BMP signalling. The Polycomb group (PcG) epigenetic axis highlights the intimate regulatory nexus between development and cancer, as its members play a critical role in the acquisition, maintenance and reversion of developmental fate [1] , whose alterations can in turn underlie the expansion or restoration of a dedifferentiated stem-like state that is thought to fuel the growth of many cancers [2] . Trimethylation of lysine 27 of histone H3 (H3K27me3), catalysed by EZH2 or EZH1 within Polycomb repressive complex 2 (PRC2), is both a major mechanism for the reversible maintenance of gene silencing [3] and one of the few histone posttranslational modifications for which bona fide evidence supports a mechanism of propagation through cell division, thus providing the molecular basis for the maintenance of aberrant repressive chromatin during cancer growth [4] . In particular, convergent lines of evidence implicate Polycomb developmental functions as critical nodes of dysregulation during tumorigenesis. First, the majority of genes that are hypermethylated in cancers on CpG promoters are pre-marked by H3K27me3 during development, corroborating the model in which PcG-dependent programmes that orchestrate normal development can be hijacked in cancer as templates for aberrant DNA methylation [5] , [6] , [7] . Second, inappropriate expression of PcG proteins was directly shown to fuel dedifferentiation [8] , and more recently the dynamic acquisition of the bivalent chromatin configuration featuring both H3K27me3 and H3K4me3, which has been associated to both embryonic and tissue-specific stem cells [9] , was found to mediate the plastic interconversion, within the same tumour, of non-cancer stem cells into cancer stem cells [10] . Furthermore, and beyond the developmental aspects of its function, the PcG system has been also implicated in other cardinal features of tumorigenesis, including silencing of the INK4A-ARF-INK4B locus [11] , promotion of angiogenesis [12] and direct control of DNA replication [13] . However, we still lack a coherent understanding of the genome-wide circuits affected by Polycomb during tumorigenesis, a deficit that has grown more relevant with accumulating evidence that PcG members can play opposing roles in tumorigenesis. Besides the ‘classical’ oncogenic properties of EZH2 (refs 14 , 15 , 16 ), recent evidence has pointed also to a tumour suppressor role manifested through either inactivating mutations of PRC2 members [17] , [18] or histone mutations that were shown to inhibit PRC2 activity [19] , [20] . Indeed, in the case of glioblastoma (GBM), although EZH2 is very frequently overexpressed, only its short-term inhibition ameliorates survival, while a longer depletion exacerbates tumour-related dedifferentiation [21] . Yet, although these results underscore the extreme context dependence of Polycomb involvement in tumorigenesis [22] , its molecular basis remains elusive. Even in settings in which EZH2 inhibition proved remarkably effective, as in lymphomas with gain-of-function mutations, it was not possible to define consistent transcriptional outputs, indicating that Polycomb can regulate different pathways even within the same apparently homogeneous tumour type [15] . This diversity of molecular impact is being linked to what is increasingly recognized, starting from Polycomb, as the core function of many chromatin modifiers, namely the definition of cell context-dependent ranges or thresholds of gene expression rather than the univocal determination of transcriptional output [2] , [23] . In turn, this grounds the rationale to pursue the elucidation of Polycomb-dependent programmes in highly defined and physiopathologically meaningful tumour models. Here we address this challenge focusing on malignant gliomas, which constitute one of the most significant unmet medical needs and present two particularly relevant features: (i) pronounced heterogeneity among and within tumour types and (ii) convergent evidence of context-dependent Polycomb involvement, which is largely limited to its impact on single genes and has not mechanistically uncovered the diversity of its target pathways in relation to specific glioma subtypes and developmental contexts [24] , [25] , [26] , [27] , [28] , [29] , [30] , [31] . Specifically, we integrate transcriptomic and epigenomic analyses to define functionally relevant PRC2-dependent networks that promote gliomagenesis, validating them both in mouse models and human samples. We find that PRC2 affects specific developmental pathways associated to defining features of the disease. Moreover, the dissection of PRC2-dependent circuits at distinct stages of gliomagenic transformation uncovers Zfp423 as a critical downstream target of PRC2, whose downregulation negatively impacts survival and whose overexpression impairs gliomagenesis in a SMAD (small mother against decapentaplegic)-dependent manner. Polycomb targets developmental pathways during gliomagenesis To define the gene circuits that are deregulated during gliomagenesis in a PRC2-dependent manner, we used a well-established mouse model of gliomagenesis that relies on the loss of Ink4a/Arf combined with the overexpression of the constitutively active mutant form of the human epidermal growth factor receptor (EGFR) known as EGFR variant III (hereafter indicated as EGFR*), the two most common lesions in human high-grade gliomas (HGGs) [32] ( Fig. 1a and Supplementary Fig. 1a ). The model relies on orthotopic transplantation of early postnatal astrocytes harbouring both lesions (hereafter Ink4a/Arf −/− ; EGFR*) and its unique advantage, as depicted in Fig. 1a , is the definition of largely homogeneous cell populations endowed with different tumorigenic potential (non-tumorigenic primary Ink4a/Arf −/− astrocytes, hereafter Astro; tumorigenic Ink4a/Arf −/− astrocytes expressing EGFR*, hereafter AstroEGFR*; glioma propagating cells (GPCs) derived from primary tumours, hereafter PT; and GPCs derived from secondary tumours, hereafter ST), which constitute a privileged entry point to dissect the transcriptional and epigenomic alterations that accrue during gliomagenesis. Importantly, the Ink4a/Arf -null background allows to study the developmental features of PRC2-dependent oncogenesis independent of its control of the INK4A-ARF-INK4B locus [11] . We first validated the model through a thorough histopathological assessment, which extended previous observations [30] , confirming that in mouse the Ink4a/Arf −/− ; EGFR* combination recapitulates a broad range of HGG, ranging from anaplastic astrocytomas, oligodendrogliomas and oligoastrocytomas to GBM and gliosarcoma ( Supplementary Fig. 1b,c ). Next, we focused on the key transition between AstroEGFR* and PT, and performed chromatin immunoprecipitation sequencing (ChIPseq) and RNA sequencing (RNAseq) for H3K27me3, to investigate the hypothesized redistribution of the PRC2 mark and its transcriptional impact during gliomagenesis. For this, we developed an ad hoc computational pipeline that integrates RNAseq and ChIPseq profiles with transcription factor (TF) motif enrichment analysis ( Fig. 1b ), to generate mechanistically testable hypotheses on the relevant Polycomb-dependent circuits. 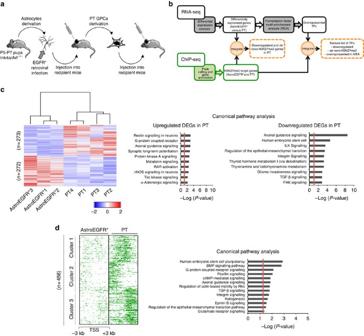Figure 1: Transcriptional changes and H3K27me3 repositioning during gliomagenesis. (a) Schematic representation of the experimental procedure followed in this study. Briefly, astrocytes derived from cortices ofInk4a/Arf−/−pups were infected with the human EGFR* and stereotaxically transplanted into recipient mice. GPCs were derived from PT and re-injected into secondary hosts to assess tumour propagation capability. (b) Schematic representation of the computational pipeline. RNAseq data were used to identify DEGs betweenInk4a/Arf−/−astrocytes overexpressing the human EGFR* (referred to as AstroEGFR*) and GPC (referred to as PT). ChIPseq data defined H3K27me3 target genes in the same cell populations. Integration of the results outlined a subset of genes that are significantly downregulated uponde novoH3K27me3 acquisition in PT. TF motif enrichment analysis (MEA) was performed on DEGs and integrated with RNAseq and ChIPseq data. (c) Left: heatmap of the DEGs between AstroEGFR* and PT. Colours representZ-scores of the row-wise normalized expression values of log2of fragments per kilobase of transcript per million mapped reads (FPKM; red: increased expression, blue: reduced expression). Right: enrichment analysis for canonical pathways in the DEGs. The probability (P-value) of random association between the gene set and given terms is calculated using the right-tailed Fisher’s exact test. Only the top ten most significant pathways are reported; bar represents the −log (P-value). (d) Left: heatmap of normalized tag densities, representing thede novomethylated genes in PT. Each row represents a 6-kb window centred on the gene TSS and extending 3 kb upstream and 3 kb downstream. The signal has been generated by merging the bam files of the biological replicates. Right: enrichment analysis for canonical pathways in the same gene set. Figure 1: Transcriptional changes and H3K27me3 repositioning during gliomagenesis. ( a ) Schematic representation of the experimental procedure followed in this study. Briefly, astrocytes derived from cortices of Ink4a/Arf −/− pups were infected with the human EGFR* and stereotaxically transplanted into recipient mice. GPCs were derived from PT and re-injected into secondary hosts to assess tumour propagation capability. ( b ) Schematic representation of the computational pipeline. RNAseq data were used to identify DEGs between Ink4a/Arf −/− astrocytes overexpressing the human EGFR* (referred to as AstroEGFR*) and GPC (referred to as PT). ChIPseq data defined H3K27me3 target genes in the same cell populations. Integration of the results outlined a subset of genes that are significantly downregulated upon de novo H3K27me3 acquisition in PT. TF motif enrichment analysis (MEA) was performed on DEGs and integrated with RNAseq and ChIPseq data. ( c ) Left: heatmap of the DEGs between AstroEGFR* and PT. Colours represent Z -scores of the row-wise normalized expression values of log 2 of fragments per kilobase of transcript per million mapped reads (FPKM; red: increased expression, blue: reduced expression). Right: enrichment analysis for canonical pathways in the DEGs. The probability ( P -value) of random association between the gene set and given terms is calculated using the right-tailed Fisher’s exact test. Only the top ten most significant pathways are reported; bar represents the −log ( P -value). ( d ) Left: heatmap of normalized tag densities, representing the de novo methylated genes in PT. Each row represents a 6-kb window centred on the gene TSS and extending 3 kb upstream and 3 kb downstream. The signal has been generated by merging the bam files of the biological replicates. Right: enrichment analysis for canonical pathways in the same gene set. Full size image A transcriptomic analysis of three independent Ink4a/ARF −/− ;EGFR* astrocyte batches along with their resulting PT led to the identification of a set of 545 differentially expressed genes (DEGs), of which 272 are downregulated and 273 upregulated in PT versus AstroEGFR*. A cluster analysis based on DEGs revealed a clear clustering by cell type (that is, with tumorigenic astrocytes segregating away from all primary tumours; Fig. 1c ). This pointed to a major and largely convergent shift in gene expression underlying the AstroEGFR*-PT transition. As shown in Fig. 1c (right), an Ingenuity Pathway Analysis (IPA) for canonical pathways uncovered the strongest enrichments among the downregulated DEGs, with a convergent involvement of genes controlling cell morphogenesis and migration, and belonging to the top scoring axonal guidance signalling, regulation of epithelial-to-mesenchymal transition (EMT) and integrin signalling pathways, whose key regulators have a well-established involvement in gliomas. Along with the related Reelin signalling pathway, axonal guidance signalling came out among the best-ranking pathways also within the upregulated DEGs ( Fig. 1c ), consistent with its dual role in regulating cell migration by fine-tuning both attractive and repulsive cues. Thus, molecules that are generally associated to repulsive clues, such as Slit2–3 and Shh , appeared to be downregulated, whereas attractors such as Wnt7b and Vegfa were upregulated, consistently with the acquisition of the infiltrating capacity that characterizes malignant gliomas. Finally, the second top-scoring enriched pathway in downregulated DEGs was human embryonic stem cell ( Fig. 1c ), whose enrichment was due to the exclusive involvement of differentiation-promoting genes. This points to dedifferentiation as a particularly significant feature of gliomagenesis and further extends the insight that gliomas originate through the reversion of either astrocytes (as in our experimental system [32] ) or neurons [33] to an undifferentiated state. Consistently, we found that Tgfb3 , known to promote neuronal differentiation [34] , Bmp4 , involved in astrocyte differentiation [35] , and Smad7 , important in neural fate acquisition [36] , were all downregulated in our PT samples. When we analysed the same cell populations for H3K27me3 distribution, comparing the number of PRC2 targets in each class of samples revealed a major overall increase of PRC2 marking in PT, with 2,306 gene hits compared with 668 in AstroEGFR*. We then compared these gene sets with two previous data sets that captured distinct aspects of PRC2 developmental control: (i) the H3K27me3 signature that characterizes cortical neural progenitors (NPs) [37] , finding that although PT samples shared a statistically significant overlap of H3K27me3 target genes with NPs (92 genes), AstroEGFR* did not show any specific overlap ( Supplementary Fig. 1e , left); and (ii) the core set of PRC2 targets whose silencing we found to be required for cell fate reversion to pluripotency [1] , finding that PT samples shared a striking overlap of H3K27me3 target genes with this core set (732 genes), whereas AstroEGFR* showed only a minimal overlap (12 genes) ( Supplementary Fig. 1e , right). Together, these results highlight the extent of developmental dysregulation and dedifferentiation that characterize this tumour model. Next, to analyse the dynamics of PRC2 targets, we focused on the 456 genes that acquire the mark during the transition from AstroEGFR* to PT consistently across all PT samples ( Fig. 1d , left). Also in this case, axonal guidance signalling and human embryonic stem cell pathways scored among the top ten in the IPA analysis of canonical pathway associated to this subset of genes ( Fig. 1d , right). Importantly, de novo targets featured three clearly distinct enrichment patterns for H3K27me3: (i) that centred on the transcription start site (TSS), with the typical pattern of great enrichment right upstream and downstream of the sharp dip coinciding with the TSS [38] ; (ii) that with a prevalent enrichment upstream of the TSS (−3 kb); or (iii) that with a prevalent enrichment downstream of the TSS (+3 kb). Comparison of expression values for genes belonging to each of the three classes showed a significant downregulation for those in which the accumulation of the mark included both the TSS and its downstream region ( Supplementary Fig. 1f ). Finally, we integrated the RNAseq and ChIPseq data sets to pinpoint the genes that, in the AstroEGFR*–PT transition, became both downregulated and de novo targets of H3K27me3 ( Fig. 2a , left). Remarkably, axonal guidance signalling was strongly associated with this subset of genes as well, indicating that this pathway is under direct Polycomb control during the gliomagenic transition ( Fig. 2a , right). 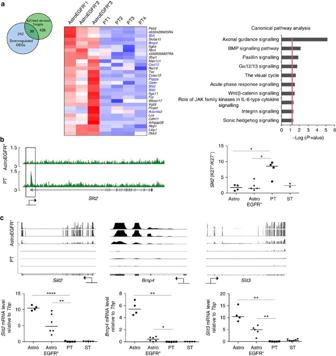Figure 2: H3K27me3-mediated downregulation affects the axon guidance pathway. (a) Left: Venn diagram displaying the overlap between downregulated DEGs (light blue) andde novoH3K27me3 targets (light green) in PT. Middle: heatmap representing the gene expression changes between AstroEGFR* and PT of the 30 downregulated DEGs andde novoH3K27me3 targets. Genes belonging to the axon guidance pathway are written in blue. Right: enrichment analysis for canonical pathways in the same gene set. (b) Left: IGV visualization of the H3K27me3 ChIPseq tracks for theSlit2gene. Black rectangle highlights the peak on the TSS. Right: ChIP–qPCR validation of the H3K27me3 enrichment. Data represent the fold increase of the K27me3-positive region of the promoter normalized on the total H3 (K27+) over a K27me3-negative region in close proximity, again normalized on the total H3 (K27−). Each symbol represents a different sample for the indicated categories on thexaxis (AstroEGFR*,Ink4a/Arf−/−astrocytes overexpressing the human EGFR*; Astro,Ink4a/Arf−/−astrocytes; PT, primary tumour GPC; ST, secondary tumour GPC); black bars within the symbols represent the median (*P<0.05) (P-values were calculated using the Mann-Whitney test). (c) Top: IGV visualization of the RNAseq tracks for selected genes of the axon guidance pathway. Bottom, analysis of transcript levels measured by qRT–PCR for the same genes. Data are represented as dCt (log2scale) relative toTbp. Each symbol represents a different sample in the specified categories on thexaxis; black bars within the symbols represent the median. (*P<0.05, **P<0.01 and ****P<0.0001) (P-values were calculated using the Mann–Whitney test). Figure 2b,c shows the independent validation of these findings for representative members of the axonal guidance signalling pathway, namely Slit2 , Slit3 and Bmp4 , which were tested for H3K27me3 enrichment ( Fig. 2b ) and expression ( Fig. 2c ). Slit2 and Slit3 are two key molecules originally involved in axon guidance (in which they provide repulsive cues by binding to their Roundabout receptors) [39] , [40] , whose functional association with glioma emerged with the observation that Slit2 is epigenetically silenced in gliomas through DNA methylation [41] , and that rescue of its expression reduces cell migration both in vitro and in vivo [42] . Bmp4 is known to reduce proliferation and promote astrogenesis [35] ; hence, its silencing further highlights dedifferentiation as a core feature of gliomagenesis. Interestingly, the core subset of genes that are both downregulated and acquire de novo H3K27me3 in the AstroEGFR* to PT transition showed a highly significant overlap with the subset of Polycomb targets that are significantly downregulated during cell reprogramming ( Supplementary Fig. 2a ). Among these genes, we found Bmp4 along with other genes involved in cellular differentiation, further emphasizing the key role played by Polycomb during the transcriptional shift from astrocytes to primary tumours ( Supplementary Fig. 2b ). Figure 2: H3K27me3-mediated downregulation affects the axon guidance pathway. ( a ) Left: Venn diagram displaying the overlap between downregulated DEGs (light blue) and de novo H3K27me3 targets (light green) in PT. Middle: heatmap representing the gene expression changes between AstroEGFR* and PT of the 30 downregulated DEGs and de novo H3K27me3 targets. Genes belonging to the axon guidance pathway are written in blue. Right: enrichment analysis for canonical pathways in the same gene set. ( b ) Left: IGV visualization of the H3K27me3 ChIPseq tracks for the Slit2 gene. Black rectangle highlights the peak on the TSS. Right: ChIP–qPCR validation of the H3K27me3 enrichment. Data represent the fold increase of the K27me3-positive region of the promoter normalized on the total H3 (K27 + ) over a K27me3-negative region in close proximity, again normalized on the total H3 (K27 − ). Each symbol represents a different sample for the indicated categories on the x axis (AstroEGFR*, Ink4a/Arf −/− astrocytes overexpressing the human EGFR*; Astro, Ink4a/Arf −/− astrocytes; PT, primary tumour GPC; ST, secondary tumour GPC); black bars within the symbols represent the median (* P <0.05) ( P -values were calculated using the Mann-Whitney test). ( c ) Top: IGV visualization of the RNAseq tracks for selected genes of the axon guidance pathway. Bottom, analysis of transcript levels measured by qRT–PCR for the same genes. Data are represented as dCt (log 2 scale) relative to Tbp . Each symbol represents a different sample in the specified categories on the x axis; black bars within the symbols represent the median. (* P <0.05, ** P <0.01 and **** P <0.0001) ( P -values were calculated using the Mann–Whitney test). Full size image Zfp423 is a master Polycomb target during gliomagenesis PRC2 had thus far been implicated in gliomagenesis on the basis of either clinical correlations [29] or of its effect on exemplary genes involved in astroglial differentiation [28] . By defining a consistent genome-wide pattern of PRC2 redistribution across independent glioma samples and characterizing its transcriptional output, our results enabled a first dissection of the specific contribution of this epigenetic axis, uncovering two prominent domains of developmental dysregulation (that is, the control of migration and differentiation outlined above). However, beyond these specific pathways and consistent with recent evidence [2] , this approach also confirmed that only a minor portion of the extensive transcriptional changes that accrue during gliomagnesis could be directly imputable to aberrant PRC2 occupancy. Thus, to gain further mechanistic insight into the functional relevance of H3K27me3 redistribution, we focused on the identification of putative PRC2-dependent master regulator TFs that could mainly and indirectly account for the transcriptional changes we observed. For this, we first performed a TF motif enrichment analysis of the DEGs between AstroEGFR* and PT. This analysis pinpointed 22 candidate master regulator TFs, defined as TFs whose binding sites were significantly enriched among the DEGs characterizing the AstroEGFR* to PT transition. These genes were then ranked according to the significance of their expression change and correlated to their H3K27me3 status. As shown in Fig. 3a , among the 22 predicted candidate master regulator TFs, Zfp423 was the only one whose repression correlated with the de novo acquisition of H3K27me3 in PT. Furthermore, meta-analysis of an RNAseq data set obtained from a different murine glioma model [21] revealed an inverse expression correlation between the PRC2 enzymatic subunit Ezh2 and Zfp423 , with Ezh2 knockdown resulting in increased Zfp423 expression ( Supplementary Fig. 3a ). We next confirmed both the downregulation ( Fig. 3b ) and the de novo H3K27me3 acquisition of Zfp423 ( Fig. 3c ) in a larger cohort of samples, highlighting the consistency of this silencing circuit. 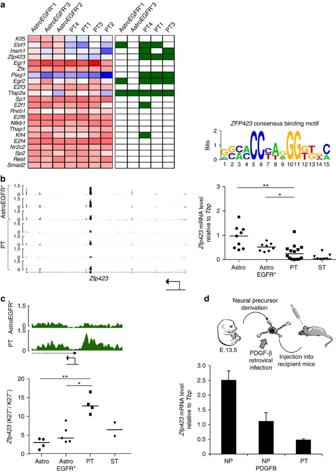Figure 3:Zfp423is downregulated in PT upon H3K27 trimethylation and its binding motif is overrepresented among DEG promoters. (a) Left: heatmap representing the gene expression levels (red: increased expression, blue: reduced expression) between AstroEGFR* and PT of the most significant, overrepresented TFs identified withPscan (BonferroniP-value<0.05). The second heatmap represents H3K27me3 status of the promoter of the same genes (white: unmethylated, green: methylated). Right:Zfp423-binding motif. (b) Left: IGV visualization of the RNAseq tracks forZfp423. Right: analysis of transcript levels measured by qRT–PCR in different cell populations. Data are represented as dCt (log2scale) relative toTbp. Each symbol represents a different sample for the specified category; black bars within the symbols represent the median. (*P<0.05 and **P<0.01) (P-values were calculated using the Mann–Whitney test). (c) Top: IGV visualization of the H3K27me3 ChIPseq tracks for theZfp423gene. Bottom: ChIP–qPCR validation of the H3K27me3 enrichment. Data represent the fold increase of the K27me3-positive region of the promoter normalized on the total H3 (K27+) over a K27me3-negative region in close proximity, again normalized on the total H3 (K27−). Each symbol represents a different sample in each category; black bars within the symbols represent the median (*P<0.05 and **P<0.01) (P-values were calculated using the Mann–Whitney test). (d) Top: schematic representation of a different glioma mouse model in whichZfp423downregulation was confirmed. Neural precursors (NPs) were isolated from telencefalic vesicles of embryos at 13.5 dpc. Cells were infected with the mousePdgf-βand transplanted stereotaxically into recipient mice. GPCs were derived from PTs. Bottom:Zfp423messenger RNA levels were measured in the different cell populations by qRT–PCR. Data are represented as dCt (log2scale) relative toTbp; error bars represent the s.d. of the technical replicates. Figure 3: Zfp423 is downregulated in PT upon H3K27 trimethylation and its binding motif is overrepresented among DEG promoters. ( a ) Left: heatmap representing the gene expression levels (red: increased expression, blue: reduced expression) between AstroEGFR* and PT of the most significant, overrepresented TFs identified with P scan (Bonferroni P -value<0.05). The second heatmap represents H3K27me3 status of the promoter of the same genes (white: unmethylated, green: methylated). Right: Zfp423 -binding motif. ( b ) Left: IGV visualization of the RNAseq tracks for Zfp423 . Right: analysis of transcript levels measured by qRT–PCR in different cell populations. Data are represented as dCt (log 2 scale) relative to Tbp . Each symbol represents a different sample for the specified category; black bars within the symbols represent the median. (* P <0.05 and ** P <0.01) ( P -values were calculated using the Mann–Whitney test). ( c ) Top: IGV visualization of the H3K27me3 ChIPseq tracks for the Zfp423 gene. Bottom: ChIP–qPCR validation of the H3K27me3 enrichment. Data represent the fold increase of the K27me3-positive region of the promoter normalized on the total H3 (K27 + ) over a K27me3-negative region in close proximity, again normalized on the total H3 (K27 − ). Each symbol represents a different sample in each category; black bars within the symbols represent the median (* P <0.05 and ** P <0.01) ( P -values were calculated using the Mann–Whitney test). ( d ) Top: schematic representation of a different glioma mouse model in which Zfp423 downregulation was confirmed. Neural precursors (NPs) were isolated from telencefalic vesicles of embryos at 13.5 dpc. Cells were infected with the mouse Pdgf-β and transplanted stereotaxically into recipient mice. GPCs were derived from PTs. Bottom: Zfp423 messenger RNA levels were measured in the different cell populations by qRT–PCR. Data are represented as dCt (log 2 scale) relative to Tbp ; error bars represent the s.d. of the technical replicates. Full size image As recounted above, gliomas display remarkable heterogeneity both at the histopathological and molecular level. In addition, we thus analysed a different mouse model that is based on the overexpression of platelet-derived growth factor beta (PDGF-B) in cortical NP (see ref. 43 and Fig. 3d ), to determine whether the glioma-associated repression of Zfp423 was consistent across different tumour-driving mutations. In this case as well, we characterized homogeneous populations of cells that captured different disease stages, namely primary, non-tumorigenic NP sourced from E13.5 telencephali (hereafter NP), tumorigenic NP overexpressing PDGF-B (hereafter NP PDGFB) and GPCs derived from primary tumours (hereafter PT) that were able to regrow tumours upon orthotopic transplantation. Consistent with our observations from the Ink4a/Arf −/− ; EGFR* model, we confirmed a progressive downregulation of Zfp423 along with the increase in tumorigenic potential ( Fig. 3d ). Zfp423 is downregulated in human gliomagenesis Although Zfp423 had not yet been associated to gliomas, a previous study [44] found the human orthologue of Zfp423 , ZNF423 , to be downregulated in human neuroblastoma. We thus assessed the expression of ZNF423 in well-defined human GBM samples that had been previously subdivided according to EGFR expression [45] and found it consistently downregulated, regardless of EGFR levels, with respect to normal human astrocytes ( Fig. 4a ), thus confirming the observation from both mouse models. We then probed a large set of clinical data available from TCGA database ( http://cancergenome.nih.gov/ ), to investigate the correlation between ZNF423 expression and patient survival. To this end, we interrogated separately low-grade gliomas and GBMs, and stratified samples according to the expression of ZNF423 . This analysis revealed a significant direct correlation between ZNF423 expression and survival in low-grade gliomas ( Fig. 4b ), with high expression associated to longer survival. The correlation held also in GBM samples, although in this more malignant subset the trend fell short of the statistical significance threshold ( Supplementary Fig. 4a ). 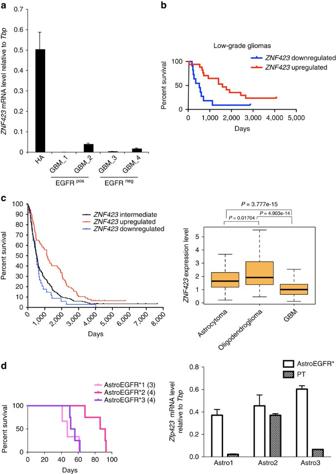Figure 4: Strong downregulation ofZfp423correlates with poor prognosis. (a) mRNA levels of the human orthologue ofZfp423,ZNF423, were measured in human glioma samples classified according to EGFR expression (GBM, GBM sample; HA, human astrocytes) by qRT–PCR. Data are represented as dCt (log2scale) relative toTBP; error bars represent the s.d. of technical replicates. (b) Kaplan–Meyer analysis of survival in low-grade glioma patients with high (red,n=17) or low (blue,n=11)ZNF423expression levels (P<0.01, data obtained from The Cancer Genome Atlas, TCGA). (c) Survival and expression analysis of a large data set from the REpository for Molecular BRAin Neoplasia DaTa (REMBRANDT). Left: Kaplan–Meyer analysis of survival in patients with high (red,n=77), intermediate (black,n=232) or low (blue,n=34)ZNF423expression levels. Difference in progression-free survival betweenZNF423high- and low-expressing patients is statistically significant (P=1.65218e−5). Right: boxplots represent expression levels ofZNF423in different samples grouped according to histopatological classification (P-values were computed with Mann–Whitney test). (d) Left: Kaplan–Meyer analysis of survival in mice injected with three representative AstroEGFR* cell lines (n=3 for AstroEGFR*1,n=4 for AstroEGFR*2 andn=3 for AstroEGFR*3). Right:Zfp423mRNA levels in the same three AstroEGFR* cell lines (white bars) and in primary GPC derived from corresponding tumours (black bars). Data are represented as dCt (log2scale) relative toTbp; error bars represent the s.d. of technical replicates. Figure 4: Strong downregulation of Zfp423 correlates with poor prognosis. ( a ) mRNA levels of the human orthologue of Zfp423 , ZNF423 , were measured in human glioma samples classified according to EGFR expression (GBM, GBM sample; HA, human astrocytes) by qRT–PCR. Data are represented as dCt (log 2 scale) relative to TBP ; error bars represent the s.d. of technical replicates. ( b ) Kaplan–Meyer analysis of survival in low-grade glioma patients with high (red, n =17) or low (blue, n =11) ZNF423 expression levels ( P <0.01, data obtained from The Cancer Genome Atlas, TCGA). ( c ) Survival and expression analysis of a large data set from the REpository for Molecular BRAin Neoplasia DaTa (REMBRANDT). Left: Kaplan–Meyer analysis of survival in patients with high (red, n =77), intermediate (black, n =232) or low (blue, n =34) ZNF423 expression levels. Difference in progression-free survival between ZNF423 high- and low-expressing patients is statistically significant ( P =1.65218e−5). Right: boxplots represent expression levels of ZNF423 in different samples grouped according to histopatological classification ( P -values were computed with Mann–Whitney test). ( d ) Left: Kaplan–Meyer analysis of survival in mice injected with three representative AstroEGFR* cell lines ( n =3 for AstroEGFR*1, n =4 for AstroEGFR*2 and n =3 for AstroEGFR*3). Right: Zfp423 mRNA levels in the same three AstroEGFR* cell lines (white bars) and in primary GPC derived from corresponding tumours (black bars). Data are represented as dCt (log 2 scale) relative to Tbp ; error bars represent the s.d. of technical replicates. Full size image In the case of neuroblastoma, ZNF423 displayed a clear trend of progressively decreased expression with more advanced tumour stages and lower expression was associated with worst prognosis. Thus, to generalize our findings and test whether ZNF423 behaved similarly in gliomas, we performed a meta-analysis of a large cohort of expression data from 343 samples of human gliomas deposited at the NCI REpository for Molecular BRAin Neoplasia DaTa [46] . As shown in Fig. 4c , we observed that also in gliomas, ZNF423 downregulation correlated with higher grade (right panel). Comparable results were obtained by performing a second meta-analysis on a further independent cohort of expression profiles, comprising 157 expression data from Gene Expression Omnibus (GEO ID: GSE4290; Supplementary Fig. 4b ). Moreover, when we classified patients from the REpository for Molecular BRAin Neoplasia DaTa database into three groups according to ZNF423 expression on the basis of their fold change with respect to median expression, a Kaplan–Meyer analysis for progression-free survival confirmed that higher levels of ZNF423 correlate with a far better prognosis compared with mid or low levels ( Fig. 4c , left panel), with high statistical significance between high- (f.c.>2) and low-expressing (f.c.<2) tumours (Mantel–Haenszel test, P =1.65218e−5). Finally, to ground the mechanistic dissection of the role of Zfp423 dosage in gliomagenesis, we resorted back to our initial Ink4a/Arf −/− ; EGFR* murine model and interrogated three independent batches of tumorigenic astrocytes (AstroEGFR*1, AstroEGFR*2 and AstroEGFR*3) with comparable Zfp423 expression. When challenged in in-vivo experiments upon orthotopic transplantation, we found that AstroEGFR*1 and AstroEGFR*3 yielded gliomas with a shorter survival compared with AstroEGFR*2 ( Fig. 4d ). Strikingly, although primary tumours originated from every astrocyte batch invariably displayed Zfp423 downregulation, they did so to different extents, with AstroEGFR*1 and AstroEGFR*3 showing a greater reduction than AstroEGFR*2 ( Fig. 4d ), thus confirming results from human data and validating this model as a sensitive system to test the physiopathologically relevant role of Zfp423 . Context-specific antigliomagenic effect of Zfp423 As higher levels of Zfp423 were associated to better prognosis in both humans and mice, we set out to validate its role by forcing its overexpression in tumorigenic Ink4a/Arf −/− ; EGFR* astrocytes and thereby test whether preventing its PRC2-mediated downregulation would impair or delay gliomagenesis. The three representative independent batches of tumorigenic astrocytes, AstroEGFR*1, AstroEGFR*2 and AstroEGFR*3, were thus infected with a retroviral vector encoding Zfp423 (ref. 47 ; hereafter AstroEGFR* Zfp423 ). Following confirmation of overexpression ( Fig. 5a ), cells were then assessed for tumorigenicity by sterotactic inoculation. Interestingly, the three AstroEGFR* lines responded differently to the challenge of Zfp423 overexpression ( Fig. 5b ). As shown in Fig. 5b , the overexpression of Zfp423 had a major impact on the tumorigenicity of AstroEGFR*2 astrocytes, with a highly statistically significant increase in survival ( P =0.0089). On the contrary, mice transplanted with either AstroEGFR*1 or AstroEGFR*3 astrocytes showed different survivals. Specifically, although AstroEGFR*1, which reached overexpression levels comparable to those in AstroEGFR*2, showed a trend of extended survival that did not reach statistical significance, AstroEGFR*3, despite much stronger Zfp423 overexpression, displayed a shorter survival. To gain insight into the molecular underpinnings of the differential response to Zfp423 overexpression, we followed two complementary approaches. 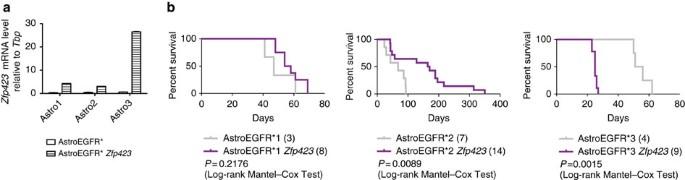Figure 5:Zfp423overexpression differentially impacts survival. (a) AstroEGFR* cell lines were infected with retroviral vectors expressingZfp423andZfp423overexpression levels were then measured by qRT–PCR. Data are represented as dCt (log2scale) relative toTbp; error bars represent the s.d. of technical replicates. (b) Kaplan–Meyer analysis of survival in mice injected with the three batches of AstroEGFR* (light grey) and AstroEGFR* overexpressingZfp423(purple). Numbers of animals for each category are indicated in brackets in the caption. Difference in progression-free survival between animals injected with AstroEGFR*2 and AstroEGFR*2Zfp423is statistically significant. Figure 5: Zfp423 overexpression differentially impacts survival. ( a ) AstroEGFR* cell lines were infected with retroviral vectors expressing Zfp423 and Zfp423 overexpression levels were then measured by qRT–PCR. Data are represented as dCt (log 2 scale) relative to Tbp ; error bars represent the s.d. of technical replicates. ( b ) Kaplan–Meyer analysis of survival in mice injected with the three batches of AstroEGFR* (light grey) and AstroEGFR* overexpressing Zfp423 (purple). Numbers of animals for each category are indicated in brackets in the caption. Difference in progression-free survival between animals injected with AstroEGFR*2 and AstroEGFR*2 Zfp423 is statistically significant. Full size image First, we performed a principal component analysis of the AstroEGFR* transcriptomes, which revealed that AstroEGFR* cluster according to their responsiveness to Zfp423 overexpression ( Fig. 6a ). Differential expression analysis uncovered gene clusters that were distinctly associated to each batch ( Fig. 6b ), which we then used to query PT transcriptomes finding that PT originated from AstroEGFR*1 and AstroEGFR*3, when compared with the AstroEGFR*2-derived PT, retained expression of a larger portion of the gene cluster belonging to the respective astrocyte batch ( Fig. 6c ). On the contrary, a shuffling analysis that randomly queried astrocyte batch-specific clusters against PT did not reveal the same degree of retention ( Supplementary Fig. 5a ). This establishes that a significant fraction of the gene expression that distinguishes similar yet distinct batches of tumorigenic astrocytes is retained in the respective tumours. Furthermore, it highlights how such tumour-retained gene expression is already primed to a greater extent in the Zfp423- resistant astrocyte batches that display, accordingly, a more aggressive tumorigenicity. This finding was strengthened by an unsupervised cluster analysis of the transcriptomes of the three AstroEGFR* and the respective PT. Indeed, each AstroEGFR* clusters with the corresponding tumour ( Supplementary Fig. 5b ), indicating that each AsroEGFR* batch is already seeded with partially specific transcriptional programmes that will unfold during tumour development. 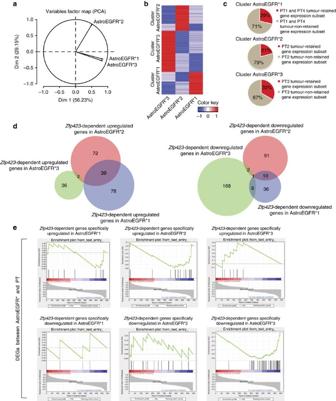Figure 6:Zfp423overexpression differentially affects AstroEGFR* networks. (a) Variable factor map (principal component analysis (PCA)) representing the degree of correlation between AstroEGFR* transcriptomes. The PCA shows that AstroEGFR* cluster according to their responsiveness toZfp423overexpression. Correlation coefficients of AstroEGFR*1, AsrtoEGFR*2 and AstroEGFR*3 with the first component are 0.8499869, 0.5120449 and 0.8380024, respectively. (b) Heatmap representing the clusters of genes selectively enriched in the three batches of tumorigenic astrocytes. (c) Pie charts representing the proportion of tumour-retained gene expression for each AstroEGFR*-derived PT. (d) Venn diagrams showing the overlap ofZfp423-dependent genes identified in the three different astrocytes batches uponZfp423overexpression. (e) Gene set enrichment analysis showing the enrichment, within the DEGs initially identified between AstroEGFR* and PT, forZfp423-dependent genes. The interrogation with theZfp423-dependent genes upregulated in AstroEGFR*2 shows a significant enrichment in the DEGs that are downregulated in the gliomagenic transition from tumorigenic astrocytes to primary gliomas. Black bars represent the position ofZfp423-dpendent genes in the ranked list of DEGs between AstroEGFR* and PT. The green line represents the enrichment score. The nominalP-values associated with theZfp423-dependent genes upregulated in AstroEGFR*2, theZfp423-dependent genes upregulated in AstroEGFR*3 and theZfp423-dependent genes downregulated in AstroEGFR*3 are statically significant (P<0.01). Figure 6: Zfp423 overexpression differentially affects AstroEGFR* networks. ( a ) Variable factor map (principal component analysis (PCA)) representing the degree of correlation between AstroEGFR* transcriptomes. The PCA shows that AstroEGFR* cluster according to their responsiveness to Zfp423 overexpression. Correlation coefficients of AstroEGFR*1, AsrtoEGFR*2 and AstroEGFR*3 with the first component are 0.8499869, 0.5120449 and 0.8380024, respectively. ( b ) Heatmap representing the clusters of genes selectively enriched in the three batches of tumorigenic astrocytes. ( c ) Pie charts representing the proportion of tumour-retained gene expression for each AstroEGFR*-derived PT. ( d ) Venn diagrams showing the overlap of Zfp423 -dependent genes identified in the three different astrocytes batches upon Zfp423 overexpression. ( e ) Gene set enrichment analysis showing the enrichment, within the DEGs initially identified between AstroEGFR* and PT, for Zfp423 -dependent genes. The interrogation with the Zfp423 -dependent genes upregulated in AstroEGFR*2 shows a significant enrichment in the DEGs that are downregulated in the gliomagenic transition from tumorigenic astrocytes to primary gliomas. Black bars represent the position of Zfp423 -dpendent genes in the ranked list of DEGs between AstroEGFR* and PT. The green line represents the enrichment score. The nominal P -values associated with the Zfp423 -dependent genes upregulated in AstroEGFR*2, the Zfp423 -dependent genes upregulated in AstroEGFR*3 and the Zfp423 -dependent genes downregulated in AstroEGFR*3 are statically significant ( P <0.01). Full size image Second, we compared by RNAseq the transcriptomes of the three batches of AstroEGFR* to their respective transcriptomes upon forced Zfp423 expression (AstroEGFR*1 versus AstroEGFR*1 Zfp423 , AstroEGFR*2 versus AstroEGFR*2 Zfp423 and AstroEGFR*3 versus AstroEGFR*3 Zfp423 ) and went on to define the Zfp423- centred transcriptional interactions specific to each pair. To this end, we integrated the results of differential expression obtained from each comparison with a co-expression-based analysis extracted from a large data set of 106 gene expression profiles collected in the GeneMania database [48] . The aim was first to infer the high confidence co-expression networks centred on Zfp423 and then define which portion of these predicted circuits were empirically validated in Zfp423 -responsive versus Zfp423 -non-responsive tumorigenic astrocytes. Consistent with the in-vivo outcome, interrogation of these gene networks showed that Zfp423 overexpression had affected different sets of genes in the three batches of tumorigenic astrocytes ( Fig. 6d ). We thus reasoned that these distinct gene subsets should display marked differences with respect to the transcriptional programme that underlies primary gliomagenesis in the same murine model. To test this hypothesis, we thus compared, by gene set enrichment analysis, the Zfp423 -dependent genes specifically affected in each batch of tumorigenic astrocyte with the DEGs that marked the AstroEGFR*-to-PT transition. This approach confirmed that the genes downregulated in the AstroEGFR*-to-PT transition were significantly enriched for the Zfp423 -dependent genes that were upregulated specifically in AstroEGFR*2, providing a clear molecular basis for the antigliomagenic effect of Zfp423 in this context. On the contrary, although we did not find any significant enrichment for Zfp423 -dependent genes affected in AstroEGFR*1, we found a significant enrichment for the Zfp423 -dependent genes affected in AstroEGFR*3, but among the genes that changed in the same direction as the DEGs characterizing the AstroEGFR*-to-PT transition ( Fig. 6e ), again providing the molecular correlate for the lack of antigliomagenic effect by Zfp423 in this context. Together, these results provide a molecular basis for the antigliomagenic impact of Zfp423 in the specific cellular context of AstroEGFR*2, grounding it in the ability to specifically antagonize a significant portion of the gliomagenesis-specific transcriptional programme that characterizes this murine model. Interestingly, among the genes specific to the Zfp423 response there are several members of the axon guidance pathways and tumour suppressor genes whose modulation was already associated to reduced tumorigenicity: namely Slit2 (refs 41 , 42 ), Pappa [49] , Nfatc4 (ref. 50 ) and Lox [51] . Furthermore, the group of genes specifically downregulated upon Zfp423 overexpression only in AstroEGFR*2 and not in AstroEGFR*1 or AstroEGFR*3 included also Sox2 and several other Sox family genes ( Supplementary Fig. 5c ), which have recently emerged as important driving or enabling factors in gliomagenesis [52] , [53] . As TF motif analysis predicted that the Sox2 promoter contains a putative binding site for Zfp423 , we asked whether Zfp423 overexpression could antagonize gliomagenesis by repressing Sox2 in Zfp423 -responsive astrocytes. To test this hypothesis, we overexpressed Sox2 in Zfp423 -responsive astrocytes to revert the phenotype of extended survival, using a construct that lacked endogenous control regions and thus could not be subjected to Zfp423 transcriptional repression. Indeed, the overexpression of Sox2 in the context of Zfp423 overexpression showed a survival rate that was much shorter compared with that achieved with Zfp423 overexpression alone ( Fig. 7a ), thus establishing Sox2 downregulation as a fundamental antigliomagenic event downstream of Zfp423 overexpression. Interestingly, however, against the expected accelerated tumorigenesis induced by overexpression of Sox2 alone, mice receiving astrocytes overexpressing both TFs showed longer survival ( Fig. 7a ), uncovering also a mutually antagonistic indirect circuit between Zfp423 and Sox2 in gliomagenesis. 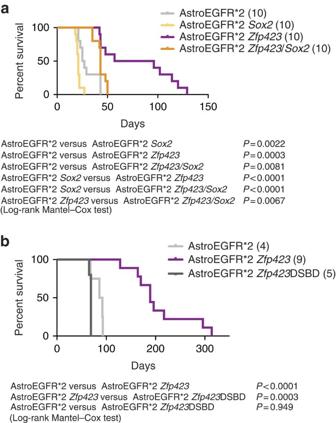Figure 7:Zfp423expression antagonizes gliomagenesis in a SMAD-dependent manner. (a) Kaplan–Meyer analysis of survival in mice injected with AstroEGFR*2 overexpressing eitherZfp423,Sox2or both. Reconstitution ofSox2expression in the context ofZfp423overexpression reverted theZfp423-dependent antigliomagenic phenotype (orange line), leading to shorter survival compared withZfp423overexpression alone (purple line). Overexpression of bothZfp423andSox2also prolonged survival with respect toSox2overexpression alone, indicating mutual antagonism between the two factors. Numbers of animals for each category are indicated in brackets in the caption;P-values were computed with log-rank Mantel–Cox test. (b) Overexpression of a mutant form ofZfp423lacking the SMAD-binding domain (Zfp423ΔSBD, dark grey curve) fails to prolong survival in mice. Numbers of animals for each category are indicated in brackets in the caption;P-values were computed with log-rank Mantel–Cox test. Figure 7: Zfp423 expression antagonizes gliomagenesis in a SMAD-dependent manner. ( a ) Kaplan–Meyer analysis of survival in mice injected with AstroEGFR*2 overexpressing either Zfp423 , Sox2 or both. Reconstitution of Sox2 expression in the context of Zfp423 overexpression reverted the Zfp423- dependent antigliomagenic phenotype (orange line), leading to shorter survival compared with Zfp423 overexpression alone (purple line). Overexpression of both Zfp423 and Sox2 also prolonged survival with respect to Sox2 overexpression alone, indicating mutual antagonism between the two factors. Numbers of animals for each category are indicated in brackets in the caption; P -values were computed with log-rank Mantel–Cox test. ( b ) Overexpression of a mutant form of Zfp423 lacking the SMAD-binding domain ( Zfp423Δ SBD, dark grey curve) fails to prolong survival in mice. Numbers of animals for each category are indicated in brackets in the caption; P -values were computed with log-rank Mantel–Cox test. Full size image Finally, in light of these analyses indicating that the Ink4a/Arf −/− ; EGFR* paradigm is more diverse than previously anticipated, we investigated this diversity considering the pronounced heterogeneity characterizing human HGG, as captured in recent molecular classifications [24] , [25] , [26] . Specifically, we used the signatures defined by Phillips et al. [24] to interrogate our cohort of PT samples and determine the extent to which they fit this classification, while measuring the spread of their molecular diversity. Notably, most murine models of glioma have not yet been interrogated with human signatures; thus, this analysis also provided a first characterization of the human equivalence, at the molecular level, of the Ink4a/Arf −/− ; EGFR* model. We found that although no PT fit neatly into either of the three categories (proneural, proliferative or mesenchymal), each encompassed different partitions of the three signatures, with a prevalence of the mesenchymal one ( Supplementary Fig. 5d ). Interestingly, most of these partitions showed opposite trends in different samples, pointing to a fundamental level of heterogeneity that accompanies, in a preferentially mesenchymal background, Ink4a/Arf −/− ; EGFR*-driven gliomagenesis. The Zfp423 antigliomagenic role engages BMP-SMAD signalling Zfp423 is widely involved in differentiation [47] , [54] , [55] , [56] , [57] , [58] , [59] , [60] . Consistently, we had previously found it greatly downregulated upon reprogramming of mouse embryonic fibroblasts into induced pluripotent stem cells [1] . Of special relevance, Zfp423 belongs also to the genes specifically expressed in the astrocyte lineage [61] , a finding that we further corroborated by inducing astrocytic differentiation and confirming the expected BMP4-enhanced upregulation of Zfp423 ( Supplementary Fig. 6a ). ZFP423 exerts its differentiation-promoting function by binding, through zinc fingers 14–20, to SMAD proteins [62] , [63] that mediate response to bone morphogenetic protein (BMP) signalling in different cell types [62] ( Supplementary Fig. 6b ). In our PT samples, both Bmp4 and Zfp423 are de novo H3K27 trimethylated and downregulated, pointing to a double and synergic blockade of the BMP signalling pathway that is critical for astroglial differentiation. Thus, also in light of the observation that Zfp423 can coordinate BMP and Notch signalling throughout neural development, and that this effect is enhanced after BMP4 stimulation [63] , we infected the Zfp423 -sensitive astrocytes (that is, AstroEGFR*2) with a well-characterized mutant isoform of Zfp423 lacking the SMAD-binding domain [47] (SBD, hereafter Zfp423 ΔSBD) and assessed their tumorigenicity in vivo . Contrary to the major antigliomagenic effect observed with the overexpression of the full-length protein, overexpression of mutant Zfp423 did not affect the tumorigenicity of AstroEGFR*2 astrocytes ( Fig. 7b ), validating the model in which the SMAD-dependent differentiating function of Zfp423 is critical for its antigliomagenic properties. HGG constitute an unmet challenge in oncology. Beyond the obvious difficulty linked to the anatomical site and the remarkable invasiveness of these tumours, two key problems have hampered progress so far: (i) the marked heterogeneity of these tumours, which implies the development of several subgroup-targeted approaches, and (ii) the virtual inaccessibility of early-stage lesions, with the attending inability to trace tumour history and define the critical gene circuits that drive initial establishment of the tumour. Notably, although many mouse models have proven invaluable in dissecting central aspects of this human disease, the experimental features of most of them precluded a thorough characterization of disease dynamics. This applies especially to the chromatin level of regulation, despite its emergence as a fundamental domain of perturbation that is raising major therapeutic hopes. Indeed, although cancer-specific chromatin maps, including for PRC2-dependent H3K27 trimethylation, are rapidly accumulating for both human and murine tumours, they most often describe endpoints of disease progression and are seldom related to transcriptional output in terms of mechanistically tested and functionally validated circuits. Here we advance significantly our understanding of PRC2 contribution to gliomagenesis with an unbiased characterization of the PRC2-dependent circuits. Specifically, we combined the informative power of a mouse model featuring homogeneous cell populations of differential tumorigenic potential with a computational pipeline for the systematic integration of RNAseq and ChIPseq profiles with discovery tools for TF motif enrichment. This yielded two key insights. First, it enabled us to functionally partition the effect of PRC2 silencing, by showing that two critical developmental domains, one centred on the morphogenetic cues that enable migration and the other centred on dedifferentiation, were under direct PRC2 control. Importantly, both have been linked to core features of HGG, such as the marked propensity for invasiveness and the aberrant re-expression of elements of the pluripotency network [33] . Second, it led to the identification of a single TF, Zfp423 , that was also under direct PRC2 control and accounted for a significant portion of the transcriptional dysregulation that underlies the transition from tumorigenic astrocytes to GPCs. Importantly, we found that Zfp423 downregulation correlated with a worse prognosis, both in two independent mouse models and in two very large cohorts of human patients. The human homologue of Zfp423 , ZNF423 , had been previously identified as a positive prognostic factor for neuroblastoma [44] ; hence, our results now extend the functional relevance of this gene to a wholly different class of tumours. The modular architecture of Zfp423 and ZNF423, whose Krüppel-like C2H2 zinc finger clusters mediate interaction with distinct transcriptional partners [62] , allowed us to mechanistically define the requirement of the BMP signalling axis for the anti-gliomagenic activity of Zfp423 , as only the full-length protein but not its SMAD mutant form was able to prolong survival. This finding is particularly interesting in light of our results demonstrating PRC2-silencing of Bmp4 in our primary tumour samples and of previous data on the aberrant recruitment of PRC2 to the BMPR1B receptor gene [28] , pointing to a synergic impact of Polycomb both on core members of the BMP signalling pathway and on one of their critical downstream effectors. Finally, our findings also uncovered a significant degree of heterogeneity within Ink4/Arf−/− ; EGFR* gliomagenesis, which we harnessed at the molecular level to define the mechanisms and context specificity of Zfp423 antigliomagenic activity. As to the former, we found that Ink4/Arf−/− ; EGFR* tumorigenic astrocytes, despite their overall similarity, display transcriptional specificities that are differentially retained in the gliomas they originate, suggesting that they represent differentially primed entry points of tumorigenesis. Consistently, this heterogeneity is carried through the primary gliomas, which encompass a relatively wide range of high-grade histopathological subtypes and also recapitulate, to different extents and for different parts, the signatures used to classify human HGG. This transcriptomic dissection of glioma heterogeneity was functionally validated with the observation that Zfp423 exerts the strongest antigliomagenic activity only in the context of the least tumour-primed astrocytes, in which it antagonizes, in an exquisitely SMAD signalling-dependent manner, a very significant portion of the gliomagenic programme that includes Sox2 , a well-established glioma oncogene, and several other differentiation-promoting factors that are specifically downregulated in gliomas. However, the context specificity displayed in this experimental model did not prevent the definition of a general prognostic impact for ZNF423 downregulation, which was confirmed in two large independent human cohorts. The context effect of Zfp423 is consistent with accumulating evidence on the extreme heterogeneity that characterizes gliomas, with a growing number of TFs being shown to play critical roles but in highly selected cases, as in the instance of the six TFs that underlie transcriptomic changes uniquely in the mesenchymal subtype HGG [26] or, even more strikingly, the FGFR-TACC oncogenic fusion that was identified in three patients from a large cohort of HGG patients [64] . Indeed, especially in light of the significant challenge posed by this remarkable heterogeneity, we believe that our approach of identifying candidate master regulators, along with their relevant networks, by comparing initiating cells with their corresponding tumours further advances the functional reclassification of gliomas on the basis of physiopathologically meaningful TF-centred pathways. Human cells Human GBM cell lines were obtained from Rossella Galli’s lab (San Raffaele Scientific Institute, Milan, Italy) and were grown as described in ref. 65 . Human astrocytes were obtained from ScienCell Research Laboratories (1810). Murine cell culture and manipulation Primary astrocytes, GPCs and NPs were derived and cultured as described previously [66] , [67] , [43] (see also Supplementary Methods ). For the astrocyte cultures, we made use of a classic protocol first descbribed in 1980. Five- to 7-day-old pups were killed, each brain was removed from the head and transferred into a cell culture dish containing sterile Dulbecco’s PBS (Lonza). Cerebral cortices were isolated from the rest of the brain and placed into a 1.5-ml tube containing 0.5 ml of astrocyte culture medium (15% North American fetal bovine serum (FBS) (Gibco), 2 mM glutamine, (Lonza), 0.6% glucose (Sigma), 100 U ml −1 potassium penicillin+100 U ml −1 streptomycin sulfate (Lonza) in basal medium Eagle’s (Gibco)). They were mechanically dissociated with scissors and through pipetting; the dissociated tissue was plated into a T-25 flask and incubated in a humidified incubator at 37 °C with 5% CO 2 . Medium was changed 3 days after plating and every other day thereafter until day 9 of culture. Cells were passaged every 4–5 days starting from day 10 of culture at a 1:2 or 1:3 ratio. The cells were rinsed with Dulbecco’s PBS and detached in trypsin–versene 1:10 (Sigma and Lonza, respectively); after detachment, the dissociation into single cells was achieved through pipetting. Trypsin was inactivated by adding FBS (Gibco, 1 volume per volume of trypsin) and cells were collected by centrifugation at 280 g for 5 min. The cell pellet was resuspended in fresh astrocyte medium and cells were plated in 6-well plates. EGFR*- or ZFP423/ZFP423dSBD-expressing retroviral particles were generated using the retrovirus producer cell line Phoenix-Eco. Established astrocyte cultures (after passage 2) were infected using the viral supernatant filtered through a 0.45-μm filter. Astrocytes were trypsinized as described before; 5 × 105 cells were resuspended in 3 ml of viral supernatant supplemented with 8 μg ml −1 Polybrene (Sigma) and plated in a well of a 6-well plate. The supernatant was removed and replaced with fresh supernatant at each new collection. Astrocytes were kept in culture for less than ten passages before being used for in-vivo experiments and next generation sequencing profiling. GPC cultures were obtained and maintained as described in Pollard et al. [67] . Mice injected with tumorigenic astrocytes were killed at the onset of neurological symptoms. The tumour mass was dissected from the brain and a small piece was put in a 1.5-ml tube containing 0.5 ml of Accutase (Sigma). The tissue was mechanically dissociated with scissors and through pipetting, passed through a 70-μm cell strainer and single cell suspension was collected in a 50-ml tube. After centrifugation (300 g for 5 min), cells were resuspended in glioma-initiating cell medium (1 × B27, 1 × N2 (Gibco), 20 ng ml −1 of both EGF and murine fibroblast growth factor-2, 100 U ml −1 potassium penicillin+100 μg ml −1 streptomycin sulfate in neurobasal medium (Gibco)) and plated in one or two wells of a six-well plate, coated with laminin (Roche). Plates were kept in a humidified incubator 37 °C with 5% CO 2 ; medium was changed 2 days after plating and every other day thereafter. Cells were passaged at 80–90% confluency at a ratio ranging from 1:3 to 1:6. They were detached with Accutase and dispersed into single cells by gentle pipetting; after centrifugation at 300 g for 5 min, cells were resuspended in glioma-initiating cell medium and plated as described above. GPCs were kept in culture for less than ten passages before being used for in-vivo experiments and next generation sequencing profiling. Differentiation was performed according to the protocol published in the same paper. In particular, astrocytic differentiation was performed by adding FBS or BMP4 to the culturing medium, whereas neuronal differentiation was achieved through growth factor withdrawal. The same protocol was used for the differentiation of embryonic neural precursors. EGFR*, Pdgf-β, Zfp423 or Zfp423DSBD retroviral particles were generated using the retrovirus producer cell line Phoenix-Eco. Supernatant was collected and used directly or after ultracentrifugation. Differentiation of NP was performed as described in ref. 67 . In vivo experiments Experiments involving animals were carried out in accordance with the Italian Laws (D.lgs. 26/2014), which enforces Dir. 2010/63/EU (Directive 2010/63/EU of the European Parliament and of the Council of 22 September 2010, on the protection of animals used for scientific purposes). Specifically, the project was notified to the Ministry of Health before the implementation of the current legislation. As the new legislation does not apply to projects approved before its enactment, for such projects only a notification of the experiments to the Ministry of Health was required (in accordance with the D.L.vo 116/92 (and following additions), which enforced EU 86/609 Directive), and this requirement was dutifully fulfilled. Tumour formation was induced by stereotaxical injection of 5 × 10 5 AstroEGFR* or GPCs into the caudate of Cd1-Nude HO, 5-week-old female mice (coordinates: 0.7 mm back, 3 mm left and 3.5 mm deep from the bregma). Brains were isolated at the onset of disease symptoms and fixed in 4% buffered formalin. Samples were paraffin embedded, sectioned, stained for haematoxylin and eosin, and histopathologically classified by pathologists. RNA and protein extraction RNA was extracted from all the lines using the RNeasy Mini Plus Kit (Qiagen) according to the manufacturer’s specifications. Quality and concentration of RNA was assessed using a NanoDropSpectrophotometer (NanoDrop Technologies). Proteins were extracted as follows: cells were harvested from the plate and centrifuged at 300 g for 5 min, then washed in PBS and lysed in RIPA buffer plus protease inhibitors cocktail (Sigma). Lysates were sonicated using the Bioruptor Sonication System (UCD200) for three cycles of 30 s with 60 s pause at high power. Lysates were centrifuged at 13,000 g for 15 min and supernatants were transferred to a new tube. Protein quantification was performed using the Bradford protein assay (BioRad) following the manufacturer’s instructions. Complementary DNA preparation and qPCR Retrotranscribed cDNAs have been obtained from 1 μg of total DNA-depleted RNA using the superscript VILO retrotranscription kit from Life Technologies according to the manufacturer’s instructions. For quantitative reverse transcriptase–PCR (qRT–PCR) analysis, a total amount of cDNA corresponding to 5 ng of starting RNA has been used for each reaction. FAST SYBR green master mix from Life Technologies and 10 μM primer pairs have been used. The qPCR reactions have been performed on an Applied Biosystems 7500 Real-Time PCR machine following the standard amplification protocol (primer list and Taqman Assays ID provided in Supplementary Tables 1 and 2 ). RNAseq and ChIPseq Library preparation for RNA sequencing was performed using RiboZero and Single Stranded kits (Illumina) according to the manufacturer’s instructions. Validation of RNAseq results has been performed through qRT–PCR analysis. For ChIPseq, cells were harvested and resuspended in PBS containing 1% formaldehyde for fixation and quenched with 125 mM glycine. Cells were lysed and sonicated using the Covaris Sonicator, to generate 250 bp DNA fragments. Chromatin was incubated overnight at 4 °C with the antibodies (H3K27me3 (Cell Signalling) and H3 total (Abcam)) and recovered the day after using Dynabeads Protein G (Life Technologies). Immunocomplexes were eluted, de-cross-linked and purified using Qiaquick PCR Columns (Qiagen) according to the manufacturer’s instructions. DNA libraries were prepared according to ChIPseq Sample Preparation Guide (Illumina) and sequenced on an Illumina GA-II or HiSeq 2000 platform. Validation of ChIPseq results has been performed through qPCR analysis: 5 ng DNA have been used for each reaction. FAST SYBR green master mix from Life Technologies and 10 μM primer pairs have been used. The qPCR reactions have been performed on an Applied Biosystems 7500 Real-Time PCR machine following the standard amplification protocol. Primer lists for qRT–PCR and ChIP–qPCR are provided in Supplementary Tables 1 and 3 . A detailed description of computational analysis is available as Supplementary Methods . Gene lists from ChIPseq and RNAseq analysis are available as Supplementary Data 1 . IPA analyses are available as Supplementary Data 2 . ChIPseq and RNAseq data have been deposited in the GEO database (GSE76292). How to cite this article: Signaroldi, E. et al. Polycomb dysregulation in gliomagenesis targets a Zfp423 -dependent differentiation network. Nat. Commun. 7:10753 doi: 10.1038/ncomms10753 (2016).